Calmodulin methyltransferase is an evolutionarily conserved enzyme that trimethylates Lys-115 in calmodulin Calmodulin (CaM) is a key mediator of calcium-dependent signalling and is subject to regulatory post-translational modifications, including trimethylation of Lys-115. In this paper, we identify a class I, non-SET domain protein methyltransferase, calmodulin-lysine N -methyltransferase (EC 2.1.1.60). A polypeptide chosen from a fraction enriched in calmodulin methyltransferase activity was trypsinized and analysed by tandem mass spectrometry. The amino-acid sequence obtained identified conserved, homologous proteins of unknown function across a wide range of species, thus implicating a broad role for lysine methylation in calcium-dependent signalling. Encoded by c2orf34, the human homologue is a component of two related multigene deletion syndromes in humans. Human, rat, frog, insect and plant homologues were cloned and Escherichia coli -recombinant proteins catalysed the formation of a trimethyllysyl residue at position 115 in CaM, as verified by product analyses and mass spectrometry. Post-translational methylation of protein lysyl residues has emerged as an important determinant of protein–protein interactions. This modification is catalysed by protein lysine methyltransferases (PKMTs), which, in conjunction with proteins with binding domains that recognize methylated lysyl residues [1] and enzymes that reverse lysyl methylation [2] , [3] , [4] , have important roles in regulating several cellular and developmental processes. Calmodulin (CaM) is a ubiquitous, calcium-dependent, eukaryotic signalling protein with a large number of interactors that is frequently trimethylated at Lys-115, a solvent-accessible residue (see PDB file 1UP5 [5] ). A limited number of studies have shown that the methylation state of CaM can change in developmental and tissue-dependent manners [6] , [7] , [8] , influence the activator properties of CaM with target enzymes [9] and cause phenotypic changes in growth and developmental processes at the level of a whole organism [10] . These observations suggest that CaM methylation could be a dynamic mechanism attenuating the interaction of CaM with target proteins influencing a plethora of eukaryotic cellular and developmental processes. The identification of the PKMTs responsible for histone methylation [11] led to our current understanding of the nuclear mechanisms that regulate gene expression and other genomic processes. The functional identification of genes for CaM lysine methyltransferase (KMT) could lead to a transformative understanding of new mechanisms regulating CaM signalling-dependent pathways in all eukaryotic organisms and highlights new roles for lysine methylation in cytoplasmic signalling pathways. The wide array of species that have protein/nucleotide sequences for CaM KMT suggests a potentially broad role for the methylation status of CaM as an important determinant of protein–protein interactions. Because of the potential importance of trimethyllysine-115 in CaM as a regulator of CaM function, we sought to provide a genetic identification of the enzyme catalysing formation of trimethyllysine-115 in CaM. After partial purification for enrichment of enzymatic activity, we identified a candidate polypeptide by photolabelling with [ 3 H-methyl] S -adenosylmethionine (AdoMet) and obtained a polypeptide sequence using tandem mass spectrometry. Homologous conserved sequences were found across a wide range of eukaryotic species, all annotated as unknown function. Using recombinant bacterial expression, we showed that these sequences encode a class I protein methyltransferase responsible for the formation of trimethyllysine in CaM. CaM KMT identification and characterization Using a previously published protocol for purification of CaM KMT [12] , we obtained a protein fraction from lamb testicles enriched ~7,500-fold in CaM KMT activity. A single Sypro ® Ruby-stained polypeptide was identified as a potential CaM KMT candidate based on molecular mass (~38 kDa) and comparison with a duplicate sample photolabelled by [ 3 H-methyl] AdoMet ( Fig. 1a ). The polypeptide was proteolysed with trypsin, and the amino-acid sequence of tryptic fragments was identified using tandem mass spectrometry (MS/MS). The deduced full-length polypeptide sequence corresponded to a protein of unknown function with a number of homologues found throughout the plant and animal kingdoms. cDNA clones from Homo sapiens ( Hs ; Isoform 1), Rattus norvegicus ( Rn ), Xenopus laevis ( Xl ), Tribolium castaneum ( Tc ) and Arabidopsis thaliana ( At ) were obtained, and after subcloning the coding regions into bacterial expression vectors, proteins were produced in Escherichia coli and the enzymes purified using bacterially expressed bovine ( Bt ) CaM-Sepharose affinity chromatography. Incubation of the recombinant enzymes with bacterially expressed forms of CaM (which lack methylation at Lys-115) in the presence of [ 3 H-methyl] AdoMet resulted in the incorporation of radiolabel into CaM ( Fig. 1b ). In vitro enzymatic assays showed that all five enzymes had robust methyltransferase activity against CaM; for example, Rn CaM KMT exhibited a k cat of 0.025 s −1 , which is comparable to the results published for CaM KMT purified to homogeneity from sheep brain (0.03 s −1 ; Fig. 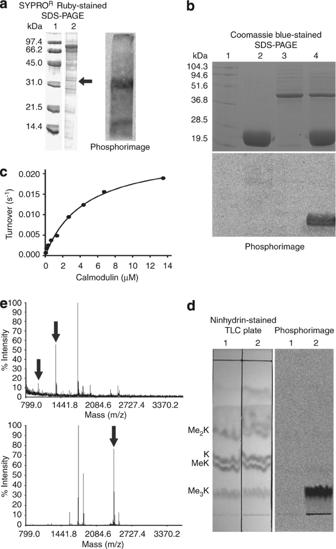Figure 1: Identification of CaM KMT. (a) Sypro®Ruby-stained SDS–PAGE (12.5%) of a lamb CaM KMT-enriched protein fraction (left panel, lane 2) and [3H-methyl] AdoMet photolabelling of an ~38 kDa polypeptide similar in molecular mass to that previously reported for the native form of CaM KMT purified to homogeneity from sheep brains12(right panel, only lane). Lane 1, molecular mass standards; (b) Coomassie blue-stained SDS–PAGE (12.5%) (top panel) and phosphorimage (bottom panel) ofRnCaMT PKMT-dependent methylation ofBtCaM. Lane 1, molecular mass standards; Lane 2,BtCaM and [3H-methyl] AdoMet, 9,950 disintegrations per min (d.p.m.) loaded; Lane 3,RnCaM KMT and [3H-methyl] AdoMet, 2,850 d.p.m. loaded; Lane 4,BtCaM,RnCaM KMT and [3H-methyl] AdoMet, 1,897,070 d.p.m. loaded; (c) Michaelis–Menten plot of turnover (s−1) versusBtCaM concentration withRnCaM KMT; (d) Thin-layer chromatographic product analyses of radiolabelled methylated lysyl residues inBtCaM after incubation with [3H-methyl] AdoMet andRnCaM KMT (Lane 2), followed by total hydrolysis in 6 N HCl. In the right panel, vertical lines define the lanes. Lane 1, standards of Lys and methylated Lys; (e) Mass spectra of trypsinizedBtCaM, unmethylated (upper panel) or after incubation withRnCaM KMT and AdoMet (lower panel). Arrows indicate masses corresponding to peptides His-107 to Lys-115 (HVMTNLGEK;m/z1,028) and Leu-116 to Arg-126 (LTDEEVDEMIR;m/z1,350) in unmethylatedBtCaM and peptide His-107 to Arg-126 (HVMTNLGE(Me3K)LT;m/z2,401), containing three methyl groups inBtCaM incubated withRnCaM KMT. 1c and Table 1 ) [12] . Figure 1: Identification of CaM KMT. ( a ) Sypro ® Ruby-stained SDS–PAGE (12.5%) of a lamb CaM KMT-enriched protein fraction (left panel, lane 2) and [ 3 H-methyl] AdoMet photolabelling of an ~38 kDa polypeptide similar in molecular mass to that previously reported for the native form of CaM KMT purified to homogeneity from sheep brains [12] (right panel, only lane). Lane 1, molecular mass standards; ( b ) Coomassie blue-stained SDS–PAGE (12.5%) (top panel) and phosphorimage (bottom panel) of Rn CaMT PKMT-dependent methylation of Bt CaM. Lane 1, molecular mass standards; Lane 2, Bt CaM and [ 3 H-methyl] AdoMet, 9,950 disintegrations per min (d.p.m.) loaded; Lane 3, Rn CaM KMT and [ 3 H-methyl] AdoMet, 2,850 d.p.m. loaded; Lane 4, Bt CaM, Rn CaM KMT and [ 3 H-methyl] AdoMet, 1,897,070 d.p.m. loaded; ( c ) Michaelis–Menten plot of turnover (s −1 ) versus Bt CaM concentration with Rn CaM KMT; ( d ) Thin-layer chromatographic product analyses of radiolabelled methylated lysyl residues in Bt CaM after incubation with [ 3 H-methyl] AdoMet and Rn CaM KMT (Lane 2), followed by total hydrolysis in 6 N HCl. In the right panel, vertical lines define the lanes. Lane 1, standards of Lys and methylated Lys; ( e ) Mass spectra of trypsinized Bt CaM, unmethylated (upper panel) or after incubation with Rn CaM KMT and AdoMet (lower panel). Arrows indicate masses corresponding to peptides His-107 to Lys-115 (HVMTNLGEK; m / z 1,028) and Leu-116 to Arg-126 (LTDEEVDEMIR; m / z 1,350) in unmethylated Bt CaM and peptide His-107 to Arg-126 (HVMTNLGE(Me3K)LT; m / z 2,401), containing three methyl groups in Bt CaM incubated with Rn CaM KMT. Full size image Table 1 Kinetic parameters for native and CaM KMT clones. Full size table CaM KMT substrate specificity Both, the degree of methylation and site specificity towards CaM, were investigated. Formation of a trimethyllysyl residue in Bt CaM was documented by product analysis after HCl hydrolysis using thin-layer chromatography and phosphorimagery after in vitro methylation with [ 3 H-methyl] AdoMet ( Fig. 1d ). Site specificity was verified using in vitro assays, followed by SDS–polyacrylamide gel electrophoresis (PAGE) and digestion of Bt CaM with trypsin and identification of peptides by MS/MS ( Fig. 1e ). The spectra included a peak at 2,401 Da, corresponding to the peptide containing Lys-115 modified by the addition of three methyl groups (42 Da) and resistant to tryptic digestion. Peptides with masses of 1,028 and 1,350 Da, products obtained from digestion in the absence of methylation, were not present in the spectra. To exclude the possibility that other lysyl residues in Bt CaM were methylated, an additional digestion of Bt CaM with Asp-N protease, followed by MS/MS peptide analyses, was performed, as the trypsin-digested methylated CaM sample had <100% coverage of lysyl-containing peptides. The spectra from both digestions confirmed that only Lys-115 was methylated. These results show that the nucleotide and associated polypeptide sequences identified here encode PKMTs specific for Lys-115 in CaM (CaM KMT; EC 2.1.1.60). CaM KMT sequence analyses All CaM KMTs contain an annotated AdoMet-binding motif found in a large number of class I methyltransferases, [13] including protein arginine methyltransferase, ribosomal protein L11 methyltransferase (PrmA) and protein isoaspartyl methyltransferase. Class I methyltransferase is known to be conserved on a defined secondary structure level, with several conserved primary sequences. Using the ESyPred3D server [14] and L11 PrmA from Thermus thermophilus as a template (2ZBQ.pdb; chain A), a molecular model for Hs CaM KMT corresponding to residues 69–292 was generated, corresponding to the catalytic domain of class I methyltransferases that bind AdoMet ( Fig. 2 ). The template, specifically chosen as a class I PKMT, shares 17.1% identity and 22.8% homology with the sequence of Hs CaM KMT ( Fig. 3 ). The N- and C-terminal regions that flank the catalytic core are predicted to possess an ordered secondary structure according to structure prediction programs, but display no sequence homology with PrmA, protein arginine methyltransferases and protein isoaspartyl methyltransferase. 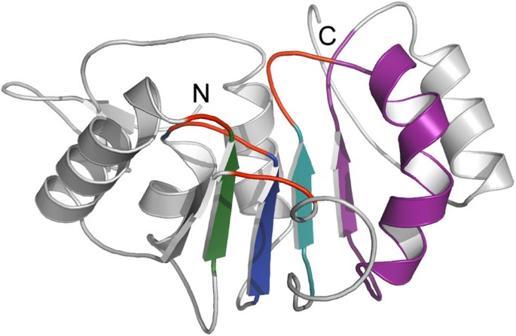Figure 2: Modelling ofHsCaM KMT as a class I MT. Molecular model of the catalytic core ofHsCaM KMT (Isoform 1) built using ESyPred3D14and based on the homology with ribosomal L11 protein lysine methyltransferase (PrmA; 2ZBQ.pdb chain A). The loops highlighted in red denote the putative AdoMet-binding site. This figure was rendered using PyMOL (http://www.pymol.org/). In the ribbon representation of the catalytic domain ofHsCaM KMT, Motif I (residues 149–158) is shown in blue, Post-Motif I (residues 174–180) in green, Motif II (residues 225–233) in teal and Motif III (residues 234–262) in purple, and are defined according to Petrossian and Clarke13. For clarity, only residues 97–291 are depicted. Figure 2: Modelling of Hs CaM KMT as a class I MT. Molecular model of the catalytic core of Hs CaM KMT (Isoform 1) built using ESyPred3D [14] and based on the homology with ribosomal L11 protein lysine methyltransferase (PrmA; 2ZBQ.pdb chain A). The loops highlighted in red denote the putative AdoMet-binding site. This figure was rendered using PyMOL ( http://www.pymol.org/ ). In the ribbon representation of the catalytic domain of Hs CaM KMT, Motif I (residues 149–158) is shown in blue, Post-Motif I (residues 174–180) in green, Motif II (residues 225–233) in teal and Motif III (residues 234–262) in purple, and are defined according to Petrossian and Clarke [13] . For clarity, only residues 97–291 are depicted. 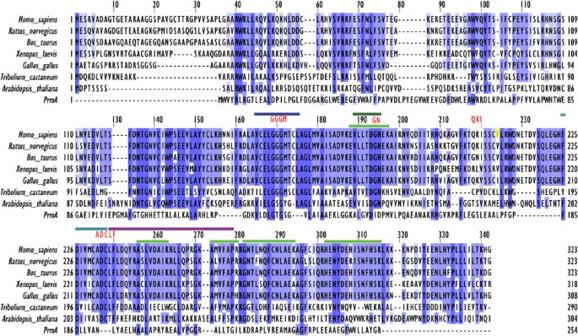Figure 3: Polypeptide sequence alignment of CaM KMTs and PrmA fromT. thermophilus. Using Jalview (www.jalview.org24), CaM KMTs and PrmA (corresponding protein accession no.AAH53733 Isoform 1, NP_001127935, NP_001099111, NP_001085547, XP_419462, XP_971600, NP_680769 and Q84BQ9, respectively) were aligned and the conservation of residues highlighted by shades of blue; the darker the colour, the more conserved the residue25. A green line over residues in the human sequence signifies the peptides that were identified by MS/MS of the partially purified lamb CaM KMT. Red letters above the human sequence are the putative residues involved in AdoMet binding based on structural comparisons with other class I MTs; the first of these represents the conserved Gly-rich loop found in all class I MTs. The yellow highlighted Phe (F) residue represents the SNP-altered residue. Amino-acid residues that correspond to Motif I, Post-Motif I, Motif II and Motif III in Class I MTs are delineated by lines coloured the same as in the model. Full size image Figure 3: Polypeptide sequence alignment of CaM KMTs and PrmA from T. thermophilus . Using Jalview ( www.jalview.org [24] ), CaM KMTs and PrmA (corresponding protein accession no.AAH53733 Isoform 1, NP_001127935, NP_001099111, NP_001085547, XP_419462, XP_971600, NP_680769 and Q84BQ9, respectively) were aligned and the conservation of residues highlighted by shades of blue; the darker the colour, the more conserved the residue [25] . A green line over residues in the human sequence signifies the peptides that were identified by MS/MS of the partially purified lamb CaM KMT. Red letters above the human sequence are the putative residues involved in AdoMet binding based on structural comparisons with other class I MTs; the first of these represents the conserved Gly-rich loop found in all class I MTs. The yellow highlighted Phe (F) residue represents the SNP-altered residue. Amino-acid residues that correspond to Motif I, Post-Motif I, Motif II and Motif III in Class I MTs are delineated by lines coloured the same as in the model. Full size image The human gene for Hs CaM KMT, c2orf34, is at locus 2p21, a region that is subject to deletions that are linked to cystinuria type I, hypotonia-cystinuria syndrome (HCS), an atypical HCS and the 2p21 deletion syndrome [15] , [16] ( Fig. 4 ). The deletions differ in size and the severity of the associated diseases correlates with the number of genes affected. Patients with atypical HCS have a deletion that spans the two genes associated with HCS (SLC3A1 and PREPL) plus c2orf34; they manifest numerous biochemical symptoms and phenotypes that are intermediate in severity between HCS and the 2p21 deletion syndrome. 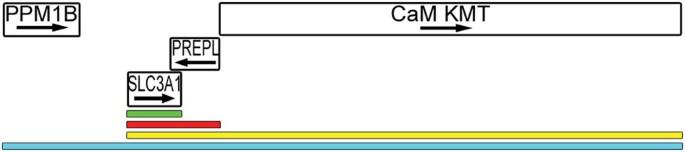Figure 4: Representation of human genes and deletions in locus 2p21 associated with different diseases. Using a screenshot ofHomo sapienschromosome 2 (GRCh37 primary reference assembly) between ~44,400 and 45,000 K nucleotides in the NCBI sequence viewer, a representation of the genes that are affected in cystinuria type I, hypotonia-cystinuria syndrome (HCS), atypical HCS and the 2p21 deletion syndrome was constructed. The boxes (gene symbol within) and the spacing between the boxes (intergenic region) are scaled appropriately. The arrow within the box represents the direction of transcription for mRNA. Coloured lines indicate the genes that are affected (by total or partial deletion) in each disease; cystinuria type I, HCS, atypical HCS and the 2p21 deletion syndrome are represented by green, red, yellow and light blue lines, respectively. These lines are not to scale regarding the size of deletions that have been characterized by two different research groups, Parvari and Creemers15,16,26,27,28. Full names of the genes according to the Human Genome Organisation are as follows: PPM1B, protein phosphatase, Mg2+/Mn2+-dependent, 1B; SLC3A1, solute carrier family 3 (cystine, dibasic and neutral amino-acid transporters, activator of cystine, dibasic and neutral amino-acid transport), member 1; PREPL, prolyl endopeptidase-like; and c2orf34, identified herein as CaM KMT, calmodulin lysine methyltransferase. Figure 4: Representation of human genes and deletions in locus 2p21 associated with different diseases. Using a screenshot of Homo sapiens chromosome 2 (GRCh37 primary reference assembly) between ~44,400 and 45,000 K nucleotides in the NCBI sequence viewer, a representation of the genes that are affected in cystinuria type I, hypotonia-cystinuria syndrome (HCS), atypical HCS and the 2p21 deletion syndrome was constructed. The boxes (gene symbol within) and the spacing between the boxes (intergenic region) are scaled appropriately. The arrow within the box represents the direction of transcription for mRNA. Coloured lines indicate the genes that are affected (by total or partial deletion) in each disease; cystinuria type I, HCS, atypical HCS and the 2p21 deletion syndrome are represented by green, red, yellow and light blue lines, respectively. These lines are not to scale regarding the size of deletions that have been characterized by two different research groups, Parvari and Creemers [15] , [16] , [26] , [27] , [28] . Full names of the genes according to the Human Genome Organisation are as follows: PPM1B, protein phosphatase, Mg 2+ /Mn 2+ -dependent, 1B; SLC3A1, solute carrier family 3 (cystine, dibasic and neutral amino-acid transporters, activator of cystine, dibasic and neutral amino-acid transport), member 1; PREPL, prolyl endopeptidase-like; and c2orf34, identified herein as CaM KMT, calmodulin lysine methyltransferase. Full size image Similar to many post-translational processing enzymes, CaM KMT is a relatively scarce enzyme. Purification of CaM KMT to homogeneity has only been accomplished once and required a purification scheme resulting in a ~20,000-fold enrichment [12] . A modified version of this protocol yielded a protein fraction ( Fig. 1a ) with high activity as a protein methyltransferase using AdoMet and Bt CaM as substrates, and enabled the identification of the protein sequences associated with CaM KMT activity across many species ( Fig. 3 ). Kinetic parameters were generally similar among CaM KMTs, with two exceptions; a higher K m for CaM for the recombinant enzymes described here compared with that reported for the native sheep brain CaM KMT and a high k cat associated with At CaM KMT ( Table 1 ). These differences could be a consequence of the different CaMs used as substrates. Previous studies relied on either naturally unmethylated forms of CaM from other species [17] or a genetically tailored and cloned form of CaM containing amino-acid sequences from both plant and vertebrate CaMs [18] . Here, we used a cloned form of bovine CaM ( Bt CaM) for Hs , Rn and Xl CaM KMT assays (because CaM is identical in mammals and amphibians), and measured At and Tc CaM KMT activity with recombinant At CaM2 and Tc CaM1, respectively. The activity of Tc CaM KMT is particularly interesting because insect CaM has been reported as unmethylated at Lys-115. Perhaps there are developmental and tissue-specific patterns to Tc CaM KMT expression that result in methylated forms of Tc CaM that have not yet been detected. CaM has been reported to be monomethylated at Lys-94 in Drosophila eyes [8] , but Tc CaM KMT only catalysed methylation of Lys-115 in our in vitro studies, as verified by MS analyses. Class I methyltransferases have signature motifs associated with the catalytic core and an AdoMet-binding site. CaM KMTs contain all of these motifs ( Figs 2 and 3 ) and also have unique C- and N-terminal flanking regions. These flanking regions may be responsible for grasping CaM and docking Lys-115 into the active site of CaM KMT for trimethylation, as is observed in the ribosomal L11 substrate-binding mode of PrmA [19] . These regions ( Hs N-terminus, Ala-38 to Asp-55, Leu-57 to Asn-69; C-terminus Leu-299, Tyr-307 to Lys-321) are also conserved across all CaM KMT homologues ( Fig. 3 ) and may show the highly conserved nature of regions involved in CaM binding. There are some annotated discrepancies with Hs CaM KMT (Isoform 1); the cDNA (accession BC053733.1 ) has a single predicted amino-acid alteration (Val-209 to Phe). However, according to amino-acid sequence alignment, the valine residue is conserved among other mammalian and amphibian CaM KMTs, and residues with similar properties are present in both insect and avian enzymes ( Fig. 3 ). Only At CaM KMT has a glutamate residue at position 209 and it is the form with the highest k cat ( Table 1 ). Although the initially expressed form of Hs CaM KMT with Phe-209 was catalytically inactive, alteration of the sequence to correspond to the gene-predicted valine restored catalytic activity to amounts similar to those observed for other CaM KMTs ( Table 1 ). To date, of the ~2,000 reported single-nucleotide polymorphisms (SNPs) for this gene, this SNP (rs17855699) has no frequency data established; thus, the significance of this discrepancy remains undetermined, although several other SNPs are apparently associated with specific human genetic backgrounds ( http://www.ncbi.nlm.nih.gov/sites/entrez?db=snp ). Several gene expression analyses suggest that there could be significant tissue-specific differences in c2orf34 expression, as well as differences between normal and cancer cell lines ( http://www.genecards.org/cgi-bin/carddisp.pl?gene=C2ORF34 ). Although Hs CaM KMT is part of two human deletion syndromes, other genes are involved ( Fig. 4 ) and a definitive assignment of a role for Hs CaM KMT in the clinical observations associated with these disorders requires further genetic analysis. However, our identification of c2orf34 as Hs CaM KMT may facilitate new genetic and biochemical approaches for further characterization of the role of Hs CaM KMT. The discovery of CaM KMT will enable a well-defined molecular and genetic approach to address whether post-translational methylation of CaM functions as a dynamic cytosolic control mechanism regulating its interaction with CaM-binding proteins, similar to the well-described effects of post-translational methylation of histones. CaM affinity column preparation A mass of 3.2 mg of unmethylated CaM ( Bt CaM) purified from bacteria (described below) was coupled to 7 ml cyanogen bromide-activated Sepharose 4 Fast Flow (Sigma Aldrich) as described by Klee and Krinks [20] . Alternatively, a pET28a Bt CaM clone, engineered to have an N-terminal His-tag, was expressed and the protein purified using HisTrap HP columns (GE Healthcare). Subsequently, recombinant Bt CaM was biotinylated using EZ-Link Iodoacetyl-LC-Biotin (Thermo Scientific) on the only cysteine within the engineered His-tag tail of this CaM and then bound to strepavidin–agarose (Millipore). CaM cloning, expression and purification Bt and Tc CaMs were cloned from a cDNA (Open Biosystems through Thermo Fisher Scientific) and from Tc cDNAs (kindly provided by Dr. S.R. Palli), respectively. The amplified sequences, after TA cloning, were subcloned to pET-28a (Novagen) and transformed into appropriate bacterial protein expression lines. Bacteria were grown at 37 °C until OD 600 reached 0.6, and were then induced with 0.5 mM isopropyl β- d -1-thiogalactopyranoside (IPTG) and collected after 4 h of additional growth at 37 °C. CaMs were purified using HisTrap HP columns (GE Healthcare), desalted by dialysis overnight, followed by treatment with a Phenyl Sepharose 6 Fast Flow column (high capacity; GE Healthcare), similar to the procedure described in Roberts et al [18] . An At CaM2 clone in a modified pET5a vector (kindly provided by Dr. R.E. Zielinski) was used for expression and the recombinant protein was purified as the other CaMs. CaM KMT partial purification Following a previously published protocol [12] , CaM KMT was partially purified from lamb testicles obtained from a local butcher shop; only the final gel filtration on Superose 12HR was omitted. [ 3 H-methyl] AdoMet photolabelling S -adenosylmethionine (AdoMet; Sigma) was purified before use [21] and diluted with [ 3 H-methyl] AdoMet (GE Healthcare) to the concentrations required in each experiment. A CaM KMT-enriched fraction was incubated with 7 μM [ 3 H-methyl] AdoMet (120×10 6 d.p.m. nmol −1 ) in 25 mM HEPES (4-(2-hydroxyethyl)-1-piperazineethanesulfonic acid; pH 7.5), 200 mM NaCl, 0.05% (w/v) CHAPS, 2 mM dithiothreitol (DTT) and 2 mM MgCl 2 on ice for 10 min. It was then transferred to a ceramic plate and crosslinked for 1 h using a 4 W UV lamp (254 nm; UVG-11 by UVP) positioned over the ceramic plate (~7 mm between the sample and the lamp). The sample was loaded on a 12.5% SDS–PAGE gel and, after electrophoresis, transferred to a PVDF membrane (Millipore) that was subsequently exposed to a storage phosphor screen (GE Healthcare) for 60 h. In-gel digestion for liquid chromatography/MSMS SDS–PAGE gel slices containing stained polypeptides were cut into 1 mm cubes, destained by two 30 min washes with 50 mM NH 4 HCO 3 /50% CH 3 CN, followed by 10 min of vortexing, then dried in a vacuum centrifuge. Proteins were reduced by addition of 50 mM NH 4 HCO 3 containing 10 mM DTT and incubation at 57 °C for 30 min. After discarding the reducing liquid, proteins were alkylated by addition of 50 mM NH 4 HCO 3 containing 50 mM iodoacetamide and incubated for 30 min in the dark at room temperature. The gel was washed twice with 50 mM NH 4 HCO 3 , once with CH 3 CN and partially dried in a vacuum centrifuge. The dried gel was rehydrated on ice for 1 h in 50 mM NH 4 HCO 3 containing 10 ng μl −1 of modified trypsin (Promega; sequencing grade). An additional 50 mM of NH 4 HCO 3 was added to cover the sample, and the gel was incubated for 18 h at 37 °C. When digested with Asp-N, the gel was rehydrated in 50 mM NH 4 HCO 3 containing 40 ng μl −1 of Asp-N and incubated immediately at 37 °C for 3–5 h. Peptides were extracted from the gel in 0.1% formic acid by sonicating for 10 min, followed by vortexing for 10 min. The extraction was repeated with 50% CH 3 CN/0.1% HCOOH, the extracts combined and the volume reduced to eliminate most of the acetonitrile. The volume of the peptide solution was adjusted to 12 μl with 0.1% HCOOH and the solution was filtered though a 0.45 μm Millex filter (Millipore) before liquid chromatography (LC)/MSMS analysis. LC/MSMS analysis Nano-flow reverse-phase LC-MS/MS was performed using a nanoLC system (Eksigent) coupled with a QSTAR XL quadrupole time-of-flight mass spectrometer (AB Sciex) through a nanoelectrospray ionization source (Protana). Analyst QS software (AB Sciex) was used for system control and data collection. The desired volume of protein solution was injected by the autosampler and desalted on a C18 trap column (300 μm×1 mm, Vydac) for 6 min at a flow rate of 10 μl min −1 . The sample was subsequently separated by a C18 reverse-phase column (75 μm×15 cm, Vydac) at a flow rate of 220 nl min −1 . The mobile phases consisted of water with 0.1% formic acid (A) and 90% acetonitrile with 0.1% formic acid (B), respectively. A 90-min linear gradient from 5 to 50% B was typically used. After LC separation, the sample was introduced into the mass spectrometer through a 10 μm silica tip (New Objective) adapted with a nanoelectrospray source (Protana). Data were acquired in information-dependent acquisition mode. Each cycle typically consisted of a 1 s time-of-flight mass spectrometry survey from 400–1,600 ( m / z ) and two 2 s MS/MS scans with a mass range of 65–1,600 ( m / z ). The LC-MS/MS data were submitted to a local MASCOT server (Matrix Science Inc.) for MS/MS ions search. CaM KMTs cloning, expression and purification The cDNA clones for Hs , Rn and Xl CaM KMT (Open Biosystems) were used as templates for amplifying the coding regions. After subcloning to pET-23b (Novagen) from pGEM-T Easy (Promega), these constructs were transformed into BL21(DE3)pLysS (Promega). Bacterial cell cultures were grown at 37 °C until OD 600 reached 0.4, and then adjusted to 0.25 mM IPTG and the culture left to grow at 20 °C for 3 h. Bacteria were lysed in 20 mM Tris (pH 8), 150 mM NaCl, 2 mM CaCl 2 , 5 mM DTT and loaded onto a Bt CaM-coupled column (prepared as described above). The column was washed extensively with 20 mM Tris (pH 8), 0.6 M NaCl, 5 mM DTT and 0.5 mM CaCl 2 , and the CaM KMTs were eluted using 20 mM Tris (pH 8), 1 M NaCl, 5 mM DTT and 1 mM EGTA. Tc and At CaM KMTs were cloned from Tc and At cDNAs that were kind gifts from Dr S.R. Palli and Dr A.B. Downie, respectively. Clones were generated in a N-terminal hexahistidine (His 6 )-Smt3 fusion vector and transformed into Rosetta(DE3)pLysS (Novagen). Bacteria were grown and induced with 0.5 mM IPTG once OD 600 reached 0.6 and the culture was left to grow overnight at 17 °C. Tc and At CaM KMT were purified using a HisTrap HP column (GE Healthcare), followed by an overnight digestion with Ulp1 protease to remove His-tag and Smt3. Finally, after affinity chromatography on a Bt CaM-coupled column as described above, the CaM KMTs were desalted by dialysis overnight and then used for kinetic assays. CaM KMT assays Using a modified protocol for Rubisco large subunit methyltransferase [22] , CaM KMT enzyme assays, in a final volume of 20 μl, were carried out using 100 mM bicine (pH 8), 150 mM KCl, 2 mM MgCl 2 , 2.5 mM MnCl 2 , 0.01% Triton X-100, 0.1 mM CaCl 2 , 2 mM DTT, [ 3 H-methyl] AdoMet (39–43 μM, 5–9×10 6 d.p.m. nmol −1 ), 0.2 μg CaM KMT and various concentrations of bacterially expressed CaM. For Hs , Rn and Xl CaM KMT assays, recombinant Bt CaM was used because CaM is identical among mammals and amphibians, whereas recombinant At CaM2 and Tc CaM1 were used for At and Tc CaM KMT assays, respectively. All reactions were performed at 37 °C for 2 min and terminated by protein precipitation with 500μl of 10% (v/v) trichloroacetic acid (TCA). The precipitated protein pellet was dissolved in 150 μl of 0.1 N NaOH and precipitated again with the same volume of TCA before dissolution in 50 μl of formic acid, followed by the addition of Bio-Safe II (Research Products International) and liquid scintillation analysis (Packard Tri-Carb 2200CA). Preparation of samples for phosphorimage analyses followed a similar protocol, except that, after the second TCA precipitation, samples were dissolved in SDS–PAGE loading buffer, electrophoresed on 12.5% SDS–PAGE gels and transferred to a PVDF membrane before exposure. Thin-layer chromatographic product analysis Bt CaM (21.6 μg) was incubated with 1 μg of Rn CaM KMT and [ 3 H-methyl] AdoMet (200 μM, 1.6×10 6 d.p.m. nmol −1 ) in a final volume of 20 μl containing 100 mM bicine (pH 8) and 20 mM MgCl 2 at 30 °C for 3 h. Because of its instability, more [ 3 H-methyl] AdoMet (same concentration as before) was added after 3 h. The volume was adjusted to 40 μl using concentrated reaction buffer to maintain the buffer strength and incubated for an additional 3 h. TCA (10% v/v) was added and the sample processed as described above for CaM KMT assays, except that the final protein pellet from TCA precipitation was subjected to complete hydrolysis with 6 N HCl, followed by analyses for methylated lysyl derivatives by thin-layer chromatography [23] . Modelling CaM KMT A molecular model of the catalytic core of Hs CaM KMT (Isoform 1) was generated on the basis of its homology with ribosomal L11 PKMT (PrmA; 2ZBQ.pdb chain A). The ESyPred3D [14] server used residues 69–292 for modelling, and the image was rendered with PyMOL ( http://www.pymol.org/ ). How to cite this article: Magnani, R. et al . Calmodulin methyltransferase is an evolutionarily conserved enzyme that trimethylates Lys-115 in calmodulin. Nat. Commun. 1:43 doi: 10.1038/ncomms1044 (2010).